Distinct structural features of TFAM drive mitochondrial DNA packaging versus transcriptional activation TFAM (transcription factor A, mitochondrial) is a DNA-binding protein that activates transcription at the two major promoters of mitochondrial DNA (mtDNA)—the light strand promoter (LSP) and the heavy strand promoter 1 (HSP1). Equally important, it coats and packages the mitochondrial genome. TFAM has been shown to impose a U-turn on LSP DNA; however, whether this distortion is relevant at other sites is unknown. Here we present crystal structures of TFAM bound to HSP1 and to nonspecific DNA. In both, TFAM similarly distorts the DNA into a U-turn. Yet, TFAM binds to HSP1 in the opposite orientation from LSP explaining why transcription from LSP requires DNA bending, whereas transcription at HSP1 does not. Moreover, the crystal structures reveal dimerization of DNA-bound TFAM. This dimerization is dispensable for DNA bending and transcriptional activation but is important in DNA compaction. We propose that TFAM dimerization enhances mitochondrial DNA compaction by promoting looping of the DNA. TFAM (transcription factor A, mitochondrial) is a multifunctional DNA-binding protein that is essential for transcriptional activation and mitochondrial DNA (mtDNA) organization [1] , [2] , [3] , [4] . As a sequence-specific transcription factor, TFAM plays a central role in production of transcripts from the light strand promoter (LSP) and the heavy strand promoter 1 (HSP1) of the mitochondrial genome. In in vitro transcription assays, normal levels of transcripts from LSP and HSP1 require TFAM [5] , [6] . These mitochondrial transcripts encode for 13 essential components of the respiratory chain, and therefore TFAM is necessary for energy production from oxidative phosphorylation [1] , [3] . In addition, TFAM is required for maintenance of mtDNA because truncated transcripts from LSP are used to prime DNA synthesis during mtDNA replication. Consistent with these functions, mice lacking TFAM have impaired mtDNA transcription and inability to maintain mtDNA, resulting in bioenergetic failure and embryonic lethality [7] . We and others have previously solved the crystal structure of TFAM bound to LSP [8] , [9] . The TFAM-binding site at LSP is 22 base pairs (bps) long and is composed of two half-sites ( Fig. 1a,b ). TFAM contains two high mobility group (HMG)-box domains (HMG-box A and HMG-box B) that each intercalates into the minor groove of a half-site. Each intercalation contributes to distortion of the DNA, resulting in a dramatic U-turn of the LSP sequence ( Fig. 1c ). Between the two HMG-box domains is a helical linker with a positively charged surface that interacts with the negatively charged backbone of the DNA. The C-terminal tail of TFAM is required for activation of the transcriptional machinery. In the TFAM/LSP structure, the carboxyl terminal HMG-box B domain binds to the half-site distal from the transcriptional start site. As the C-terminal tail is adjacent to the HMG-box B, the U-turn in the LSP DNA enables the C-terminal tail to contact the transcriptional machinery. Consistent with this idea, TFAM mutants that are deficient in DNA bending are inactive for transcriptional activation at LSP [8] . In contrast, the same mutants are fully active at HSP1. On the basis of sequence comparisons, TFAM has been suggested to bind to HSP1 in the reverse orientation compared with LSP [10] , [11] . We proposed that in this reverse orientation, the C-terminal tail would be located near the half-site adjacent to the transcriptional machinery, rendering DNA bending unnecessary [8] . However, this model hinges on the expectation that the TFAM is indeed reversed on HSP1 compared with LSP, an idea that lacks experimental evidence. 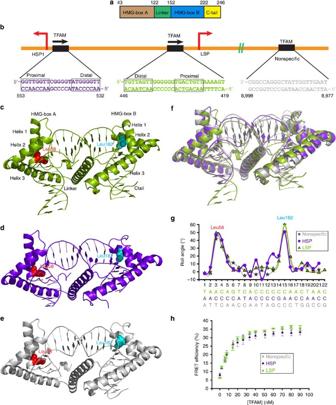Figure 1: Overview of the TFAM–mtDNA complexes. (a) The domain structure of mature TFAM. Residues 1–42 constitute the mitochondrial targeting sequence that is cleaved upon the import of TFAM into the mitochondrial matrix. (b) Schematic of DNA sequences bound within TFAM crystals. Note the different orientations of TFAM on LSP versus HSP1. The nonspecific sequence is from theATPase6gene. The half-sites of LSP and HSP1 are indicated. (c–e) Side view of the TFAM/LSP, TFAM/HSP1 and TFAM/nonspecific DNA complexes, respectively. The major intercalating residues, Leu58 and Leu182 are highlighted. The DNA fragments are colour-coded as inb. (f) Superimposition of TFAM crystal structures, colour-coded as inb. (g) Comparison of roll angle values for TFAM/LSP, TFAM/HSP1 and TFAM/nonspecific DNA. Note that there are two peaks of DNA distortion, at the positions where Leu58 and Leu182 intercalate. (h) FRET assay for DNA bending with three different DNA templates: LSP, HSP1 and nonspecific DNA. Data points are the average of three independent experiments, with error bars representing s.d.’s. Figure 1: Overview of the TFAM–mtDNA complexes. ( a ) The domain structure of mature TFAM. Residues 1–42 constitute the mitochondrial targeting sequence that is cleaved upon the import of TFAM into the mitochondrial matrix. ( b ) Schematic of DNA sequences bound within TFAM crystals. Note the different orientations of TFAM on LSP versus HSP1. The nonspecific sequence is from the ATPase6 gene. The half-sites of LSP and HSP1 are indicated. ( c – e ) Side view of the TFAM/LSP, TFAM/HSP1 and TFAM/nonspecific DNA complexes, respectively. The major intercalating residues, Leu58 and Leu182 are highlighted. The DNA fragments are colour-coded as in b . ( f ) Superimposition of TFAM crystal structures, colour-coded as in b . ( g ) Comparison of roll angle values for TFAM/LSP, TFAM/HSP1 and TFAM/nonspecific DNA. Note that there are two peaks of DNA distortion, at the positions where Leu58 and Leu182 intercalate. ( h ) FRET assay for DNA bending with three different DNA templates: LSP, HSP1 and nonspecific DNA. Data points are the average of three independent experiments, with error bars representing s.d.’s. Full size image TFAM has an equally important function in organization of the mitochondrial genome. Located in the mitochondrial matrix and lacking histone-related proteins, mtDNA is organized into compact mtDNA/protein structures termed nucleoids [12] , [13] . TFAM is one of the most abundant proteins of the nucleoid [14] , [15] and is thought to coat the entire mitochondrial genome and compact it [16] , [17] . On the basis of the TFAM/LSP structure, it is tempting to assume that TFAM also imparts a U-turn when bound nonspecifically to mtDNA. In this manner, TFAM would shorten the apparent length of the mitochondrial genome by coating it and imposing regular sharp bends. The structurally unrelated HU family of proteins also imparts U-turns on DNA and may play an analogous role in the architecture of prokaryotic genomes [18] , [19] . However, it is unclear whether the structure of TFAM bound to LSP, where it binds in a sequence-specific mode, serves as a good model for TFAM coating the mitochondrial genome, where it functions as a nonspecific DNA-binding protein. Although TFAM bends DNA at LSP, it has been suggested that such rigid DNA bends are not applicable when TFAM is bound to nonspecific DNA [20] . Moreover, it remains to be determined whether DNA bending is a sufficient mechanism to account for the dramatic condensation of mtDNA within a nucleoid compared to naked circular DNA. In this study, we present additional crystal structures of TFAM bound to HSP1 and to nonspecific mtDNA, and show that in both cases TFAM imposes a U-turn on the DNA. We experimentally confirm that TFAM binds HSP1 in the opposite orientation compared with the TFAM/LSP structure and provide evidence that this orientation difference underlies the different requirements of the two promoters for DNA bending. In the four existing TFAM structures, we observe dimerization of TFAM via the same protein–protein interface. We show that dimerization is not needed for DNA bending or transcriptional activation but is necessary for full compaction of DNA. These results suggest that TFAM dimerization provides an additional compaction mechanism beyond DNA bending to help organize mtDNA into nucleoids. Comparison of TFAM bound to specific and nonspecific DNA We previously solved the crystal structure of TFAM bound to its cognate-binding site on LSP [8] ( Fig. 1a–c ). This structure indicates that TFAM imposes a U-turn on LSP DNA upon binding; however, the generality of this observation is unknown. It is unclear whether the TFAM/LSP structure is representative of how TFAM binds to HSP1, where DNA bending by TFAM is dispensable for transcriptional activation [8] . Even more important, it is unclear whether TFAM also imparts a U-turn when it binds nonspecific mtDNA, where it is thought to play an important role in DNA packaging. To address these issues, we generated crystal structures of TFAM bound to HSP1 mtDNA and nonspecific mtDNA. Our initial attempt to generate such structures yielded small and poorly diffracting crystals. As the TFAM/LSP structure indicates that the last nine residues of TFAM are disordered [8] , [9] , we repeated crystallization trials with a new TFAM construct (residues 43–237) lacking these disordered residues. We obtained well-diffracting crystals of TFAM bound to a 22-bp double-stranded DNA fragment from HSP1 ( Fig. 1d ; termed the TFAM/HSP1 structure). This DNA fragment contains the TFAM-binding site determined by DNAse I footprinting [21] . In addition, we crystallized TFAM in complex with a 22-bp fragment from the ATPase6 gene as an example of TFAM binding nonspecifically to mtDNA ( Fig. 1e ; termed the TFAM/nonspecific DNA structure). Both the TFAM/HSP1 and TFAM/nonspecific DNA structures were solved by molecular replacement using the coordinates of TFAM/LSP [9] as the search model. The structures of TFAM/HSP1 and TFAM/nonspecific DNA were solved at a resolution of 2.9 Å and 2.8 Å, respectively. For both, the final electron density maps were of sufficient quality to visualize all the protein residues and the entire DNA fragment. Model building and refinement led to final R work and R free values of 22.55% and 26.53% for TFAM/HSP1, and 21.37% and 26.11% for TFAM/nonspecific DNA, respectively. Details of the crystallographic analyses are presented in Table 1 . Table 1 Data collection and refinement statistics. Full size table The TFAM/HSP1 and TFAM/nonspecific DNA structures are highly similar to TFAM/LSP [8] , [9] . Superimposition against the TFAM/LSP structure generates RMSD values of 1.056 Å for TFAM/HSP1 and 0.951 Å for TFAM/nonspecific DNA ( Fig. 1f ). In each case, TFAM binding imposes a full U-turn on the DNA. This U-turn is caused by the wedging of the two HMG-box domains of TFAM into the minor groove of the DNA. Each HMG-box domain consists of three helices that are arranged in an L-shaped configuration stabilized by hydrophobic interactions ( Fig. 1c–e ). The concave surface of each HMG-box domain intercalates into the DNA minor groove, with contributions from Leu58 and Ile81 of HMG-box A and Asn163, Pro178 and Leu182 of HMG-box B ( Fig. 1c–e , Supplementary Fig. 1 ). Analysis of DNA parameters indicates that distortion of the DNA double helix is maximal at the bases contacted by Leu58 and Leu182 ( Fig. 1g ). A helical linker with a positively charged surface connects the two HMG-box domains and packs against the overlaying DNA [8] , [9] . As originally described for TFAM/LSP, the two intercalating HMG-box domains and the linker, acting as a pivot, work in concert to impart a U-turn on the bound DNA. TFAM imposes a U-turn regardless of mtDNA sequence Taken together, these crystal structures indicate that TFAM bends DNA into a U-turn, whether bound specifically to LSP or HSP1, or bound nonspecifically to a random mtDNA fragment. To determine whether this DNA distortion also occurs in solution, we used an established Förster resonance energy transfer (FRET)-based assay to measure DNA bending [8] . To construct the FRET sensor, Cy3 (donor) and Cy5 (acceptor) fluorophores were covalently attached to opposite ends of the LSP, HSP1 and ATPase6 (nonspecific) DNA fragments. Addition of TFAM to the labeled, double-stranded DNA resulted in a dose-dependent increase in acceptor emission and a decrease in donor emission. Control experiments confirmed that the acceptor emission depended on the presence of both the donor fluorophore and TFAM. For each DNA fragment, the maximal FRET efficiency corresponds to a calculated distance of 59 Å between the DNA ends, in good agreement with the distances in the crystal structures (TFAM/LSP: 54.7 Å; TFAM/HSP1: 53.7 Å; TFAM/nonspecific DNA: 52.9 Å; Fig. 1f,h ). These data indicate that all three DNA templates are bent to a similar degree by TFAM, suggesting that the formation of U-shaped DNA is relevant not only in transcriptional activation but also in mtDNA packaging. Reverse binding orientations of TFAM to LSP and HSP1 On the basis of DNA sequence analysis of the promoters, TFAM has been proposed to bind in opposite orientations on LSP versus HSP1 (refs 10 , 11 ). This idea has implications about the mechanism of transcriptional activation by TFAM, and therefore it is important to obtain direct experimental support. To unambiguously assign the orientation of the DNA sequence in the TFAM/HSP1 structure, we substituted thymine at position 550 with bromo-uracil ( Fig. 2a,b ). This substitution uniquely labels HSP1 DNA at the half-site proximal to the transcriptional initiation site. Bromine has significant anomalous scattering signal, and X-ray data from isomorphous crystals showed an anomalous peak (>5σ) at the expected position for bromine adjacent to the HMG-box B domain ( Fig. 2c,d ). These data confirm that TFAM binds HSP1 with HMG-box B occupying the proximal half-site, the orientation opposite to that found in the TFAM/LSP complex. 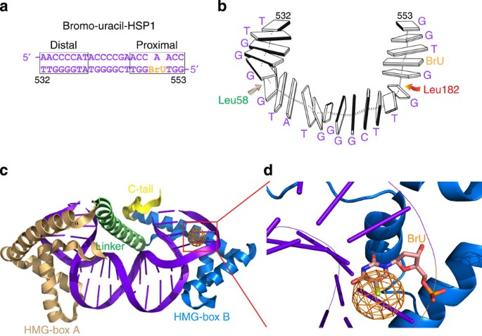Figure 2: TFAM binds HSP1 in a reverse orientation. (a) The labeled DNA template used to determine the orientation of TFAM on HSP1. Thymine 550 was replaced with bromo-uracil to label the proximal half-site. (b) A presentation of the 22 bp HSP1 structure, showing its U-turn shape and the location of intercalating residues. (c) The TFAM/HSP1 complex showing location of the anomalous signal of bromo-uracil (orange) relative to the domains of TFAM. The anomalous signal is adjacent to HMG-box B. (d) Close-up view of the anomalous electronic density in a Friedel-pair difference map revealing a >5σ peak (orange). Figure 2: TFAM binds HSP1 in a reverse orientation. ( a ) The labeled DNA template used to determine the orientation of TFAM on HSP1. Thymine 550 was replaced with bromo-uracil to label the proximal half-site. ( b ) A presentation of the 22 bp HSP1 structure, showing its U-turn shape and the location of intercalating residues. ( c ) The TFAM/HSP1 complex showing location of the anomalous signal of bromo-uracil (orange) relative to the domains of TFAM. The anomalous signal is adjacent to HMG-box B. ( d ) Close-up view of the anomalous electronic density in a Friedel-pair difference map revealing a >5σ peak (orange). Full size image We analysed the interaction of TFAM to the DNA bases in each of the three structures ( Supplementary Fig. 2 ). Interestingly, the TFAM/LSP structure shows several additional base contacts that are absent in the TFAM/HSP1 and TFAM/nonspecific DNA structures. These additional contacts, mediated by Gln179 and Arg157, may explain why TFAM makes a robust, discrete DNAse I footprint on LSP DNA [21] . We did not observe additional base contacts in TFAM/HSP1 compared with TFAM/nonspecific DNA. DNAse I footprinting studies indicate that TFAM has lower specificity for HSP1 relative to LSP. At TFAM concentrations that result in protection of the HSP1 site, the surrounding DNA is also coated [21] . We used in vitro transcription reactions with LSP or HSP1 templates to test the idea that different structural features of TFAM are required for activation of these promoters. Transcription from the LSP and HSP1 promoters can be reconstituted in vitro by providing the DNA templates with mitochondrial RNA polymerase, TFB2M and TFAM [5] . We previously generated a mutant (L6) that contained point mutations (K136A, H137A, K139A, R140A, K146A and K147A) in the helical linker connecting the two HMG-box domains of TFAM [8] . This mutant showed the most severe DNA-bending defect from a panel of mutants. Like other DNA-bending mutants, L6 is defective in activating transcription from LSP ( Supplementary Fig. 6B ). However, this mutant is able to activate transcription at HSP1 as effectively as wild-type TFAM [8] ( Fig. 3b,c ). 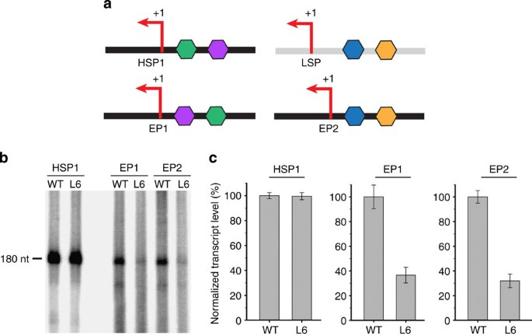Figure 3: Conversion of HSP1 into a promoter dependent on DNA bending. (a) Schematics of HSP1, LSP and two engineered promoters (EP1 and EP2) derived from HSP1. EP1 and EP2 were designed to reverse the orientation of TFAM on HSP1. (b) Representative transcription reactions with wild-type TFAM and the L6 mutant that is deficient in DNA bending. (c) Quantification of transcription reactions, with error bars representing s.d.’s from three independent experiments. Values are normalized to that of wild-type TFAM. Figure 3: Conversion of HSP1 into a promoter dependent on DNA bending. ( a ) Schematics of HSP1, LSP and two engineered promoters (EP1 and EP2) derived from HSP1. EP1 and EP2 were designed to reverse the orientation of TFAM on HSP1. ( b ) Representative transcription reactions with wild-type TFAM and the L6 mutant that is deficient in DNA bending. ( c ) Quantification of transcription reactions, with error bars representing s.d.’s from three independent experiments. Values are normalized to that of wild-type TFAM. Full size image To probe the basis for this defect, we asked whether HSP1 could be converted into a promoter that is sensitive to DNA bending by TFAM. In the first approach, we reversed the TFAM-binding site at HSP1, so that HMG-box B would now bind at the distal half-site ( Fig. 3a , EP1 template). In the second approach, we replaced the TFAM-binding site in HSP1 with the corresponding region from LSP, again forcing TFAM to bind in a reverse orientation compared with native HSP1 ( Fig. 3a , EP2 template). When tested with in vitro transcription assays, both these modified HSP1 promoters are activated by wild-type TFAM. However, the bending defective L6 mutant shows a several-fold decrease in transcriptional activation ( Fig. 3b,c ). Dimerization of TFAM Along with the two new TFAM structures reported here, there are now four structures of TFAM bound to DNA. Remarkably, all the structures reveal dimerization of TFAM stabilized by an identical dimer interface. In each case, the dimer interface occurs between HMG-box A of two separate TFAM molecules. HMG-box A consists of three helices arranged in an L-shape, with helix 3 forming the long edge. 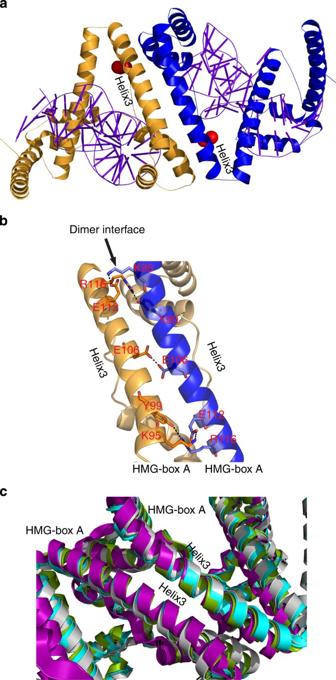Figure 4: Dimerization interface. (a) Overview of two molecules of TFAM forming a dimer in the TFAM/HSP1 crystal structure. Each TFAM molecule is bound to its own DNA fragment. Helix 3 from one HMG-box A domain forms an antiparallel interface with the corresponding helix 3 from another molecule. The locations of the cysteines used for protein labeling are indicated in red. (b) Close-up of the antiparallel dimerization interface. Residues involved in hydrogen bonds and salt bridges are labeled. (c) Superimposition of the dimerization interfaces from all four TFAM/DNA structures: TFAM/LSP—28 bp (green, pdb:3TMM), TFAM/LSP—22 bp (cyan, pdb:3TQ6), TFAM/HSP1—22 bp (purple) and TFAM/nonspecific DNA—22 bp (grey). RMSD values relative to TFAM/LSP—22 bp are as follows: TFAM/LSP—28 bp, 0.887; TFAM/HSP1—22 bp, 1.056; TFAM/nonspecific DNA—22 bp, 0.951. Figure 4a shows the interface found within the asymmetric unit of TFAM/HSP1. The convex surfaces of two HMG-box A domains come into contact, with helix 3 from each domain paired in an antiparallel manner ( Fig. 4a ). The antiparallel interface shows a series of polar and electrostatic interactions mainly mediated by residues Lys95, Tyr99, Glu106, Glu112 and Arg116 of helix 3 ( Fig. 4b ). In the helix 3/helix 3 interface, Lys95 forms a salt bridge with Glu112, and Tyr99 forms a hydrogen bond with Arg116. Between helices 3 and 1, Arg116 interacts with Glu63, and Glu106 interacts with Arg59. With over 30 residues involved, the dimer interface has a total buried surface area of ~1,179 Å 2 ( Supplementary Fig. 1B ). In the TFAM/LSP 22 bp (ref. 9 ), TFAM/LSP 28 bp (ref. 8 ) and TFAM/nonspecific DNA structures, the generation of symmetry mates from the asymmetric unit reveals identical, antiparallel helical interfaces that superimpose well on the interface found in TFAM/HSP1 ( Fig. 4c ). This interface is unrelated to the C-terminal region previously proposed as a candidate dimerization motif [17] . Figure 4: Dimerization interface. ( a ) Overview of two molecules of TFAM forming a dimer in the TFAM/HSP1 crystal structure. Each TFAM molecule is bound to its own DNA fragment. Helix 3 from one HMG-box A domain forms an antiparallel interface with the corresponding helix 3 from another molecule. The locations of the cysteines used for protein labeling are indicated in red. ( b ) Close-up of the antiparallel dimerization interface. Residues involved in hydrogen bonds and salt bridges are labeled. ( c ) Superimposition of the dimerization interfaces from all four TFAM/DNA structures: TFAM/LSP—28 bp (green, pdb:3TMM), TFAM/LSP—22 bp (cyan, pdb:3TQ6), TFAM/HSP1—22 bp (purple) and TFAM/nonspecific DNA—22 bp (grey). RMSD values relative to TFAM/LSP—22 bp are as follows: TFAM/LSP—28 bp, 0.887; TFAM/HSP1—22 bp, 1.056; TFAM/nonspecific DNA—22 bp, 0.951. Full size image TFAM dimerization is not required for DNA bending or transcriptional activation To test the physiological function of dimerization, we generated a TFAM mutant with five substitutions (K95A, Y99F, E106A, E112A and R116A; hereafter termed ‘dimer mutant’) designed to disrupt polar and electrostatic interactions at the interface. These five residues in the dimerization interface are conserved in mammals ( Supplementary Fig. 3 ). To assess TFAM dimerization, we developed a FRET-based assay to measure TFAM/TFAM contact. We covalently labeled TFAM molecules with either a donor fluorophore (Alexa Fluor 488) or an acceptor fluorophore (Alexa Fluor 595) using cysteine–maleimide chemistry at the single cysteine residue at position 49 ( Fig. 4a ), which is close to the dimer interface. In the absence of DNA, no FRET was detected between the two labeled populations (red trace, Fig. 5a ). However, in the presence of DNA, we found a decrease in donor emission and an increase in acceptor emission (magenta trace, Fig. 5a ). This FRET signal could be competed off by excess unlabeled TFAM ( Supplementary Fig. 4A ). This FRET signal was abolished in the dimer mutant (blue trace, Fig. 5a , Supplementary Fig. 4B ), suggesting loss of dimerization. Interestingly, the dimerization of wild-type TFAM was not only dependent on DNA, but also on the length of the DNA. Testing a range of DNA lengths (100, 150, 200, 300 to 400 bp), we found robust TFAM dimerization only with DNA fragments ≥200 bps ( Fig. 5b ). 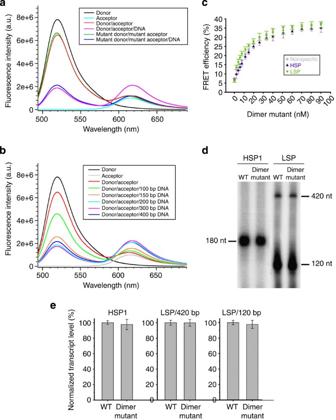Figure 5: Biochemical analysis of TFAM dimerization. (a) Emission spectra in a FRET assay measuring the physical interaction between TFAM molecules. Reactions contained Alexa Fluor 488 (donor)-labeled and/or Alexa Fluor 594 (acceptor)-labeled TFAM. Fluorescence emission spectra showed FRET signal only in the presence of plasmid DNA (magenta trace). Note that this signal was abolished in the dimer mutant (blue trace). (b) Emission spectra of wild-type TFAM incubated with linear DNA of varying lengths. (c) DNA bending by the dimer mutant on three templates. Data points are the average of three independent experiments, with error bars representing s.d.’s. (d) Representative transcription assay using wild-type TFAM or the dimer mutant. The LSP template generates a 420 nt full-length (run-off) transcript and a truncated 120 nt transcript. (e) Quantification of transcription reactions with error bars representing s.d.’s from three independent experiments. Figure 5: Biochemical analysis of TFAM dimerization. ( a ) Emission spectra in a FRET assay measuring the physical interaction between TFAM molecules. Reactions contained Alexa Fluor 488 (donor)-labeled and/or Alexa Fluor 594 (acceptor)-labeled TFAM. Fluorescence emission spectra showed FRET signal only in the presence of plasmid DNA (magenta trace). Note that this signal was abolished in the dimer mutant (blue trace). ( b ) Emission spectra of wild-type TFAM incubated with linear DNA of varying lengths. ( c ) DNA bending by the dimer mutant on three templates. Data points are the average of three independent experiments, with error bars representing s.d.’s. ( d ) Representative transcription assay using wild-type TFAM or the dimer mutant. The LSP template generates a 420 nt full-length (run-off) transcript and a truncated 120 nt transcript. ( e ) Quantification of transcription reactions with error bars representing s.d.’s from three independent experiments. Full size image Although defective in dimerization, the dimer mutant has normal secondary structure ( Supplementary Fig. 5 ) and is fully functional for DNA binding ( Supplementary Fig. 6A ) and bending on LSP, HSP1 or nonspecific DNA templates ( Fig. 5c ). Moreover, the dimer mutant is as efficient as wild-type TFAM in transcriptional activation from either the LSP or HSP1 template ( Fig. 5d,e ). Taken together, these data suggest that dimerization is dispensable for both DNA bending and transcriptional activation. DNA bending and TFAM dimerization are required for efficient DNA compaction In addition to transcriptional activation, the other major function of TFAM is mtDNA compaction. In the latter function, TFAM is thought to interact with mtDNA in a global, nonspecific manner. To analyse the ability of TFAM mutants to compact DNA, we utilized a tethered particle motion (TPM) assay ( Fig. 6a ), in which the contour lengths of single DNA molecules are measured upon interaction with TFAM [22] , [23] . In this assay, one end of a DNA molecule is attached to a bead, and the other end is immobilized on a slide. Because the DNA molecule has a defined length, the tethered bead will have a characteristic radius of motion that can be quantified as a root-mean-square (RMS) value. Addition of TFAM to the system reduces the radius of motion by decreasing the end-to-end length of the DNA tether, a reflection of DNA compaction ( Fig. 6a ). Using a 1,910-bp DNA tether, we found progressively lower RMS values with increasing TFAM concentrations ( Fig. 6b ). The naked DNA tether had an RMS value of 295 nm; this value was reduced to 164 nm under saturating TFAM concentrations (1 μM). By testing a panel of DNA lengths ranging from 539 to 1,910 bp, we found that TFAM at saturating concentration reduces the apparent lengths proportionally to the original length of the tether ( Fig. 6c ). To compare these DNA compaction effects, we generated a DNA calibration curve for naked DNA ( Supplementary Fig. 7A ). This calibration curve allowed us to convert RMS values in the presence of TFAM to apparent DNA length, and thereby calculate the extent of compaction in terms of base pairs ( Supplementary Fig. 7B ). Regardless of the original DNA length, TFAM shortened the DNA contour-length by 64–73% ( Fig. 6d ). 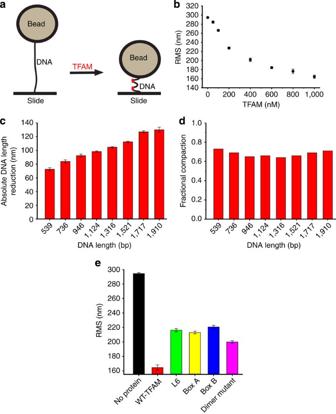Figure 6: Structural determinants of DNA compaction. (a) A schematic of the TPM assay. The bead is attached by a single DNA molecule to the glass surface. Upon addition of TFAM, the contour length of the DNA molecule is reduced, causing a decrease in the bead’s radius of motion. (b) Effect of increasing concentrations of TFAM on the DNA contour length. A 1,910-bp DNA fragment was used. Error bars indicate s.e.m. from three independent experiments. (c) DNA compaction by TFAM on DNA fragments of varying lengths. Error bars represent s.e.m. from three independent experiments. (d) Fractional shortening of DNA by TFAM as a function of DNA length. (e) Maximal DNA compaction by wild-type TFAM and mutants. A 1,910-bp DNA fragment was used. Error bars illustrate s.e.m. from three independent experiments. Figure 6: Structural determinants of DNA compaction. ( a ) A schematic of the TPM assay. The bead is attached by a single DNA molecule to the glass surface. Upon addition of TFAM, the contour length of the DNA molecule is reduced, causing a decrease in the bead’s radius of motion. ( b ) Effect of increasing concentrations of TFAM on the DNA contour length. A 1,910-bp DNA fragment was used. Error bars indicate s.e.m. from three independent experiments. ( c ) DNA compaction by TFAM on DNA fragments of varying lengths. Error bars represent s.e.m. from three independent experiments. ( d ) Fractional shortening of DNA by TFAM as a function of DNA length. ( e ) Maximal DNA compaction by wild-type TFAM and mutants. A 1,910-bp DNA fragment was used. Error bars illustrate s.e.m. from three independent experiments. Full size image This level of DNA compaction exceeds the maximal shortening that can be accounted for by DNA bending and prompted us to examine the structural basis for DNA compaction in the TPM assay. In the TFAM crystal structures, a 22-bp DNA fragment is shortened by ~50% because of formation of a U-turn. Multiple regions of TFAM are important for bending mtDNA [8] , [9] , including both HMG-box domains and the intervening helical linker. Using the 1,910-bp DNA tether, we compared the compaction abilities of TFAM mutants previously established as having a DNA-bending defect [8] . While wild-type TFAM compacted DNA molecules to 164 nm, TFAM truncation mutants containing either HMG-box A alone or HMG-box B alone shortened DNA to only 212 nm and 227 nm, respectively ( Fig. 6e ). The linker region of TFAM coordinates the spacing and orientation of the two HMG-box domains and is important for DNA bending. The L6 linker mutant also shows a defect in DNA compaction. Hence, both HMG-box domains as well as the intervening linker are necessary to achieve efficient DNA compaction. This result is not surprising, given that an important aspect of DNA compaction should be the formation of DNA U-turns. To examine whether TFAM dimerization might affect DNA compaction, we tested the dimer mutant in the TPM assay. We found that the dimer mutant has a substantial defect in DNA compaction, with an RMS value of 193 nm ( Fig. 6e ). This DNA compaction defect is not due to loss of DNA binding because the mutant binds to DNA with the same affinity as wild-type TFAM ( K d ~6–7 nM, Supplementary Fig. 6A ) and has no defect in either DNA bending or transcriptional activation ( Fig. 5c–e ). These results therefore uncover TFAM dimerization as an important aspect of DNA compaction. Our study provides several important insights into the structural biology of TFAM. First, by providing additional TFAM structures, we show that TFAM imposes a U-turn on mtDNA whether it is bound at LSP, HSP1 or nonspecific DNA. Therefore, extreme DNA bending is a constitutive feature of TFAM binding. It has been suggested that DNA U-turns may not be relevant when TFAM is bound to nonspecific DNA [20] . However, we show that TFAM mutants defective in bending have a reduced ability to compact nonspecific DNA. Second, we provide evidence that the different orientations of the TFAM-binding sites at LSP compared with HSP1 underlie the different sensitivities of these promoters to the DNA-bending activity of TFAM ( Fig. 7a,b ). At LSP, the C-terminal tail is oriented away from the transcriptional start site, and a U-turn in the DNA is required to bring the C-terminal tail in contact with the transcriptional machinery ( Fig. 7a ). At HSP1, we directly confirmed by bromine-labeling that the TFAM orientation is reversed. This new orientation places the C-terminal tail close to the transcriptional machinery and negates the need for DNA bending ( Fig. 7b ). This model is further supported by promoter engineering experiments where we converted HSP1 into a DNA-bending-dependent promoter by reversing the TFAM orientation. Finally, we found that the four existing TFAM/DNA structures show dimerization of TFAM with an identical interface formed by HMG-box A/HMG-box A interactions. In our previous study, we ignored this interface as a potential crystal-packing artifact; however, its presence in four independent structures makes this explanation unlikely. Using a FRET assay, we detected a TFAM–TFAM interaction that is strictly dependent on the presence of DNA. Analysis of the dimer mutant indicates that dimerization is not required for DNA bending or transcriptional activation at LSP or HSP1. However, the TFAM dimer mutant shows substantially reduced DNA compaction in a TPM assay. Taken together, these results suggest that specific structural features of TFAM are critical, depending on the specific function. At LSP, DNA bending at the promoter is central to transcriptional activation, whereas at HSP1, this feature is dispensable. TFAM dimerization plays a key role in mtDNA compaction but not in transcriptional activation. 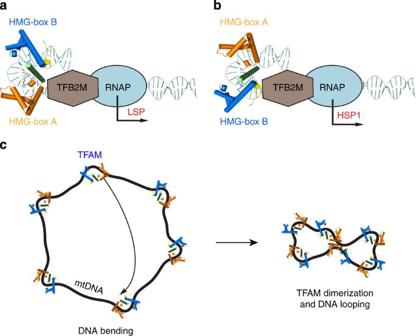Figure 7: Models of transcription activation by TFAM and mtDNA packaging. (a,b) Comparison of TFAM function on LSP versus HSP1. When bound on LSP (a), TFAM is oriented with the HMB-box B domain binding the distal half-site. As a result, the U-turn in DNA is necessary to position the C-terminal tail (small yellow region) towards the transcriptional machinery. The C-terminal tail is essential for transcriptional activation10and physically interacts with TFB2M45, but additional interactions with mtRNA polymerase are also possible. When bound to HSP1 (b), TFAM is oriented with the HMG-box B domain binding the proximal half-site. The C-terminal tail is positioned close to the transcriptional machinery, and DNA bending is dispensable for transcriptional activation. (c) Model of mtDNA compaction. Upon binding to mtDNA, each TFAM molecule imposes a local U-turn. When TFAM coats mtDNA, the formation of multiple U-turns results in mtDNA compaction. In addition, TFAM monomers can dimerize through the HMG-box A domain. This interaction forms DNA loops, which further compact mtDNA in the nucleoid. Figure 7: Models of transcription activation by TFAM and mtDNA packaging. ( a , b ) Comparison of TFAM function on LSP versus HSP1. When bound on LSP ( a ), TFAM is oriented with the HMB-box B domain binding the distal half-site. As a result, the U-turn in DNA is necessary to position the C-terminal tail (small yellow region) towards the transcriptional machinery. The C-terminal tail is essential for transcriptional activation [10] and physically interacts with TFB2M [45] , but additional interactions with mtRNA polymerase are also possible. When bound to HSP1 ( b ), TFAM is oriented with the HMG-box B domain binding the proximal half-site. The C-terminal tail is positioned close to the transcriptional machinery, and DNA bending is dispensable for transcriptional activation. ( c ) Model of mtDNA compaction. Upon binding to mtDNA, each TFAM molecule imposes a local U-turn. When TFAM coats mtDNA, the formation of multiple U-turns results in mtDNA compaction. In addition, TFAM monomers can dimerize through the HMG-box A domain. This interaction forms DNA loops, which further compact mtDNA in the nucleoid. Full size image A recent study showed that single TFAM molecules can extensively slide over nonspecific DNA [20] . Some sliding monomers of TFAM were observed to collide with immobile TFAM multimers and aggregate into patches. Combined on our crystallographic analysis, it appears that even though TFAM enforces a severe bend on nonspecific DNA, it can nevertheless slide long distances. During transcription, this sliding may allow the RNA polymerase to migrate through TFAM-coated mtDNA. In future work, it will be interesting to determine whether the TFAM multimers utilize the dimerization motif we have identified. Our results suggest that two factors—DNA bending and TFAM dimerization—are involved in mtDNA compaction. In the TFAM/DNA structures, the formation of a U-turn compresses the 22-bp recognition sequence by ~50% end-to-end. This extreme DNA bending requires spatial coordination of the tandem HMG-box domains by the helical linker. TFAM variants containing a single HMG-box domain or mutations in the helical linker show defective DNA bending and, in the TPM assay, reduced DNA compaction. Although DNA bending is clearly important, it alone cannot account for the 64–73% compaction that we observed in the TPM assay. Based on the behaviour of the dimer mutant, this additional compaction appears to require TFAM dimerization. Given that the TPM assay measures the effective length of individual DNA tethers, this dimerization occurs between TFAM molecules bound to a single DNA fragment. TFAM dimerization in solution is only observed with DNA templates ≥200 bps in length, probably because dimerization of TFAM molecules bound on the same DNA fragment would lead to DNA looping ( Fig. 7c ), a phenomenon that is constrained by the persistence length of DNA. In contrast, under the high protein/DNA concentrations used for crystallography, dimerization was observed between TFAM molecules bound to separate, short DNA fragments. Some other DNA looping proteins have been reported to condense DNA to a much greater extent [24] , [25] than we have found for TFAM. It is likely that the TFAM dimerization is weak, and at equilibrium, there is a balance between dimerization and dissociation that results in a moderate degree of compaction from this mechanism. It should be noted that the type of dimerization implied by our results is distinct from the dimerization suggested in previous studies. Some studies have suggested that TFAM binds to a single DNA-binding site as a dimer [17] , [26] . This mode of binding is unlikely, given the multiple crystal structures showing that the TFAM-binding sites identified by DNAse I footprinting are fully occupied by a single TFAM molecule. The idea that a TFAM monomer binds to DNA is further supported by multi-angle light scattering [8] and single molecule measurements [20] . These findings clarify the mechanism for mtDNA packaging by TFAM. One aspect involves iterations of mtDNA bending caused by coating of the genome by TFAM. Measurements in tissues [16] , [27] and cells [28] , [29] suggest that TFAM is abundant enough to fully coat the mitochondrial genome. Moreover, recombinant TFAM can coat nonspecific DNA in vitro with an occupancy of one molecule per ~30 bp (ref. 20 ), close to the theoretical maximum based on a minimal TFAM-binding site of 22 bp. The repeated application of DNA bending would cause significant shortening of the end-to-end length of a DNA molecule. This condensed DNA molecule can be further compacted by TFAM dimerization, which would result in looping of the DNA between bound sites. Dimerization can only occur between TFAM molecules spaced the appropriate distance apart. In principle, the 16-kb mtDNA genome is long enough to accommodate many potential loops. However, in our dimerization assay, we do not observe a linear increase in the FRET signal as the DNA length is increased, suggesting that there may be unknown constraints. Interestingly, atomic force microscopy images of DNA compacted in vitro by TFAM show the formation of DNA loops consistent with this model [17] . TFAM purification and labeling Full-length, mature human TFAM (43–246), TFAM lacking the last nine residues (43–237), and mutants were expressed and purified as hexahistidine fusion proteins [8] . The hexahistidine tag was removed with thrombin cleavage. The proteins were further purified using gel filtration chromatography using a Hi-load Superdex 200 16/60 column (GE Healthcare) pre-equilibrated with running buffer (20 mM Tris-HCl, 300 mM NaCl, 1 mM dithiothreitol (DTT), pH 7.5) in an AKTA Purifier (Amersham). The protein was concentrated to 20 mg ml −1 and stored at −80 °C. To obtain fluorescently labeled TFAM, recombinant TFAM (43–237), containing only a single reactive cysteine at position 49, was incubated with either Alexa Fluor 488 maleimide or Alexa Fluor 595 maleimide (Molecular Probes) [30] . The protein was dialysed in buffer (50 mM HEPES, pH 7.5, 350 mM NaCl), diluted to 0.1 mM and treated with 0.5 mM TCEP ( tris (2-carboxyethyl)phosphine) for 90 min at 4 °C to ensure reduction of cysteine residues. The labeling reaction was carried out using a sixfold excess of Alexa Fluor maleimide for 15 h at 4 °C and stopped by 3 mM DTT. Unreacted dye was removed with a 15-cm desalting column (Sephadex G-25 Medium, GE Healthcare). The concentration of labeled protein was determined by absorbance of Alexa Fluor 488 ( ε 495 =73,000 M −1 cm −1 ) and Alexa Fluor 595 ( ε 590 =92,000 M −1 cm −1 ). The labeling efficiency (moles of labeled protein per moles of total protein) was typically ≥95%. Crystallization and structure determination The duplex HSP1 DNA was generated by mixing complementary oligonucleotides: 5′-GGTT 550 GGTTCGGGGTATGGGGTT-3′; 5′-AACCCCATACCCCGAACCAACC-3′. The nonspecific mtDNA template was generated by mixing complementary oligonucleotides: 5′-ATTCAACCAATAGCCCTGGCCG-3′; 5′-CGGCCAGGGCTATTGGTTGAAT-3′. For the bromine derivative of the HSP1 duplex, thymine 550 of HSP1 was substituted with bromo-uracil (5′-GGT/i5Br-dU/GGTTCGGGGTATGGGGTT-3′) (Integrated DNA Technologies, San Diego) and annealed with its non-labeled complementary strand. To form the TFAM (43–237)/HSP1 or TFAM (43–237)/HSP1-Br complexes, 0.57 mM TFAM was mixed with 0.65 mM duplex DNA in a 1:1 volume ratio, incubated at room temperature for 30 min and then on ice for 2 h. Crystallization trials by hanging drop-vapour diffusion at room temperature identified conditions (12% PEG8000, 22% glycerol, 0.04 M KH 2 PO 4 , pH 6.0) that yielded plate-shaped crystals. To form the TFAM (43–237)/nonspecific DNA complex, 0.57 mM TFAM was mixed with 0.65 mM duplex DNA in a 1:1 volume ratio, incubated at room temperature for 30 min and then on ice for 3 h. For crystallization trials, the protein/DNA complex was mixed with reservoir solution in a 1.2:0.8 volume ratio. The complex was crystallized by hanging drop-vapour diffusion at room temperature (9% PEG1500 and 18% glycerol), yielding plate-shaped crystals. Crystals were flash-frozen in liquid nitrogen, and diffraction data of both native and bromo derivative crystals were collected on beamline 12-2 at the Stanford Synchrotron Radiation Lightsource. The data set from the TFAM/HSP1-Br crystal was collected at the Br-absorption peak (0.9196 Å). To avoid radiation damage, diffraction data from a second TFAM/HSP1-Br crystal were collected at native wavelength (1.0332 Å), and this diffraction data set was used for the final refinement. A crystal of the TFAM/nonspecific DNA complex was collected at 0.9795 Å. All data were processed with IMOSFLM [31] or XDS [32] and merged using SCALA [33] as implemented in CCP4. The two structures were solved by molecular replacement using the coordinates of the TFAM/LSP crystal structure [9] . The electron density map revealed clear density for the protein and DNA. The bromine derivative of TFAM/HSP1 yielded anomalous signal that allowed unambiguous assignment of the DNA sequence. Manual model building was carried out in COOT [34] , and refinement of the best solutions was carried out using REFMAC [34] and PHENIX [35] with an initial round of rigid body refinement followed by a round of simulated annealing and individual B-factor refinement. After a few rounds of model adjustment and refinement with TLS obtained from the TLSMD server [36] , the R work converged to 22.11% and R free to 26.74% for TFAM/HSP1-Br, and 21.37 and 26.11% for TFAM/nonspecific DNA. A stereo image of a portion of the final electron density is provided in Supplementary Fig. 8 . The final models include residues 43–237 of TFAM, and all the nucleotides have excellent stereochemistry as assessed by MolProbity [37] . The Ramachandran plots reveal that 94.1% and 97.9% allowed regions with no outliers for TFAM/HSP1-Br and TFAM/nonspecific DNA, respectively. Analyses of the helical parameters of the DNA molecules were carried out using 3DNA [38] . Structural superimpositions and figures were prepared with Chimera 1.5.2 (ref. 39 ), COOT [34] , PyMol [40] , 3DDART [41] and NUCPLOT [42] . FRET experiments for DNA bending To generate the LSP, HSP1 and nonspecific DNA templates, the following complementary oligonucleotides were annealed as described above: LSP: 5′/Cy3/-TGTTAGTTGGGGGGTGACTGTTAAAAGT-3′; 5′/Cy5/-ACTTTTAACAGTCACCCCCCAACTAACA-3′; HSP1: 5′/Cy3/-GGTTGGTTCGGGGTATGGGGTT-3′; 5′/Cy5/-AACCCCATACCCCGAACCAACC-3′; nonspecific: 5′/5Cy5/-ATTCAACCAATAGCCCTGGCCG-3′; 5′/5Cy3/-CGGCCAGGGCTATTGGTTGAAT-3′. Annealing reactions were performed with a small excess of acceptor-labeled DNA relative to donor-labeled DNA (1.2:1 molar ratio) to ensure that all donor-labeled DNA had a paired acceptor DNA strand [43] . For FRET analysis [8] , [43] , measurements were recorded on a FluoroMax-3 spectrofluorimeter (Jobin–Yvon–Horiba) at room temperature. Protein was titrated into a cuvette containing either 10 nM Cy3-labeled, Cy5-labeled or Cy3-Cy5-labeled DNA in binding buffer (20 mM Tris (pH 7.5), 150 mM NaCl, 1 mM DTT). For all the mutants, the protein titrations were carried out to at least 10-fold in excess of the K d for DNA binding. Excitation wavelengths for Cy3 and Cy5 are 525 nm and 625 nm, respectively; emission wavelengths are 562 and 662 nm. For Cy3- or Cy3-Cy5-labeled DNA, scans were recorded using excitation at 525 nm and emission from 540 to 750 nm. For Cy5-labeled DNA, scans were recorded with excitation at 625 nm and emission from 640 to 750 nm. Slit widths for excitation and emission were 4 nm and 10 nm, respectively. The FRET efficiency ( E ) was calculated with the following formula: E =( F corr )/( F corr + D corr ), where F corr =[ F –( χ D D )−( χ A A )]/ σ A and D corr = D / σ D . F corr =corrected FRET fluorescence; D corr =corrected fluorescence from donor alone; D =donor fluorescence; A =acceptor fluorescence; χ D =donor bleed-through coefficient; χ A =acceptor coefficient. σ A and σ D are measured correction factors for acceptor and donor fluorescence, respectively, as defined below. In FRET measurements, the signals due to donor bleed-through ( χ D ) and direct excitation of acceptor ( χ A ) need to be corrected. χ D and χ A were determined by using the DNA fragment labeled with only a single fluorophore. To determine χ D , Cy3-labeled DNA was excited at 525 nm, and emissions were collected at 562 nm ( D ) and 662 nm ( F ). χ D =( F/D ). To calculate χ A , Cy5-labeled DNA was excited at 525 nm ( F ) or 625 nm ( A ), and emissions were collected at 662 nm. χ A =( F/A ). We also corrected for changes in fluorescence intensity between the unbound and bound species. For the donor signal, the correction factor σ D was calculated by dividing the donor signal of bound DNA (b) by the donor signal of unbound DNA (u) using Cy3-labeled DNA. σ D = D b / D u . For the acceptor signal, σ A was calculated by dividing the acceptor signal of bound DNA by the acceptor signal of unbound DNA using Cy3-Cy5-labeled DNA. σ A = A b / A u . The distance ( R ) between donor and acceptor pairs was calculated from the following equation: E = R 0 6 /( R 0 6 + R 6 ), where E =FRET efficiency and R 0 =54 Å. FRET measurements to detect dimerization To detect dimerization of TFAM through the HMG-box A domain, Cys49 in HMG-box A was labeled with either Alexa Fluor 488 or Alexa Fluor 595 (see above). Fluorescence measurements were recorded on a FluoroMax-3 spectrofluorimeter (Jobin–Yvon–Horiba) at room temperature (20 mM Tris-HCl (pH 7.5), 150 mM NaCl and 1 mM DTT). Alexa Fluor 595-labeled protein (400 nM) was added to 100 nM Alexa Fluor 488-labeled protein in the presence and absence of DNA. DNA tested included fragments of various lengths (100, 150, 200, 300 and 400 bp) and circular plasmid (4 kb). When the experiment was performed with DNA, 10 nM of linear DNA, or 1 nM of circular plasmid DNA, was added to the mixture containing both TFAM labeled with Alexa Fluor 488 and Alexa Fluor 594. The acceptor fluorescence signal could be chased off with excess non-labeled wild-type protein. The signal was monitored by excitation at 480 nm, and emission spectra were recorded from 494 to 690 nm. Slit widths for excitation and emission were 4 nm and 10 nm, respectively. In vitro transcription reactions DNA fragments corresponding to LSP (positions 1–477) and HSP1 (positions 499–741) of human mtDNA were cloned into the pSP65 vector at the Bam HI and Sal I sites. EP1 was constructed by reversing the TFAM-binding site at HSP1, and EP2 was made by subcloning the TFAM-binding site from LSP into HSP1. LSP: 5′-A 454 AAT AATGTGTTAGTTGGGGGGTGACTGTT AAAA 421 -3′; HSP1: 5′-T 528 GCT AACCCCATACCCCGAACCA ACC AAAC 557 -3′; EP1: 5′-T 528 GCT TGGTTCGGGGTATGGGGTT AGC AAAC 557 -3′; EP2: 5′-T 528 GCT AATGTGTTAGTTGGGGGGTGACTGTT AAAC 557 -3′. The engineered promoters were synthesized by PCR with the appropriate oligonucleotides and cloned into the pSP65 vector at the Bam HI and Sal I sites. After digestion with Bam HI for LSP and Sal I for HSP1 derivatives, the linearized plasmids were used as templates in a transcriptional run-off assay [8] . Transcription reactions were performed in a total volume of 20 μl (10 mM HEPES (pH 7.5), 10 mM MgCl 2 , 1 mM DTT, 100 μg ml −1 bovine serum albumin (BSA), 400 μM ATP, 150 μM rCTP, 150 μM rGTP, 15 μM rUTP (Promega), 0.2 μM [α- 32 P] rUTP (3,000 Ci mmol −1 , Perkin Elmer), 7.5 nM template DNA and 40 units of RNaseOut (Invitrogen)). Reactions were carried out at 33 °C by incubating the template DNA with buffer for 5 min, then subsequently adding TFAM (100 nM), TFB2M (30 nM, Enzymax) and POLRMT (30 nM, Enzymax), with 1 min incubations between each addition. After addition of rNTPs, the reaction was incubated for 3 h at 33 °C and stopped by addition of 25 μl of stop buffer (80% formamide, 10 mM EDTA, pH 8.0, 0.025% xylene cyanol and 0.025% bromophenol blue). Samples were heated to 90 °C for 5 min and separated on 5% polyacrylamide gels containing 8 M urea in 1 × Tris/borate-EDTA buffer. The gels were fixed in 7% acetic acid, dried and exposed to a phosphorimager screen. The data were collected on a Storm 880 phosphorimager (Molecular Dynamics) and quantified using the ImageQuant 5.2 Software. TPM assays The TPM assay [22] , [23] was used to measure DNA compaction. Non-sequence-specific DNA molecules of different lengths (539, 736, 946, 1,124, 1,316, 1,521, 1,717 and 1,910 bp) were assembled in a flow cell between a glass surface and a bead. These DNA molecules were immobilized by attaching the 5′-digoxigenin-labeled DNA to a glass surface coated with anti-digoxigenin (Roche Diagnostics). The other end of the DNA was attached to a 490-nm streptavidin-coated polystyrene bead (Bangs Laboratories) via a 5′-biotin label. The flow cell surface was passivated with acetylated-BSA and casein to prevent the DNA, beads and protein of interest from sticking. The motion of the bead was recorded through a brightfield microscope at 30 frames per second using a Basler A602f camera. Fits were performed using custom Matlab routines [44] . At least 20 single DNA tethers were measured in buffer containing 20 mM Tris-HCl, pH 7.5, 1 mM DTT, 150 mM NaCl and 100 μg ml −1 A-BSA. Circular dichroism analysis All circular dichroism data were collected on an Aviv 62DS spectrometer with a 1-mm path length cell. The protein sample of wild-type TFAM and the dimer mutant was 10 μM in 20 mM Tris-HCl (pH 7.5), 300 mM NaCl and 1 mM DTT. Far-UV circular dichroism spectra were collected at 25 °C, with a data-averaging time of 5 s. The data were collected every 1 nm from 195 to 260 nm. DNA-binding measurements The TFAM DNA-binding assay measures the quenching of intrinsic tryptophan fluorescence that occurs when TFAM binds DNA. Measurements were recorded on a FluoroMax-3 spectrofluorimeter (Jobin–Yvon–Horiba) at room temperature (20 mM Tris-HCl (pH 7.5), 150 mM NaCl and 1 mM DTT). DNA was titrated into a cuvette containing 50 nM protein. The solution was monitored by excitation at 280 nm, and emission spectra were recorded from 320 to 380 nm. Slit widths for excitation and emission were 4 nm and 10 nm, respectively. The binding data were analysed using the SigmaPlot 9.0 software. Accession codes: Coordinates and structure factors for the TFAM/Br-HSP1 DNA and TFAM/nonspecific DNA crystal structures have been deposited in the Protein Data Bank under accession numbers 4NOD and 4NNU . How to cite this article: Ngo, H. B. et al. Distinct structural features of TFAM drive mitochondrial DNA packaging versus transcriptional activation. Nat. Commun. 5:3077 doi: 10.1038/ncomms4077 (2014).